Sustained Wnt/β-catenin signalling causes neuroepithelial aberrations through the accumulation of aPKC at the apical pole β-Catenin mediates the canonical Wnt pathway by stimulating Tcf-dependent transcription and also associates to N-cadherin at the apical complex (AC) of neuroblasts. Here, we show that while β-catenin activity is required to form the AC and to maintain the cell polarity, oncogenic mutations that render stable forms of β-catenin (sβ-catenin) maintain the stemness of neuroblasts, inhibiting their differentiation and provoking aberrant growth. In examining the transcriptional and structural roles of β-catenin, we find that while β-catenin/Tcf transcriptional activity induces atypical protein kinase C (aPKC) expression, an alternative effect of β-catenin restricts aPKC to the apical pole of neuroepithelial cells. In agreement, we show that a constitutively active form of aPKC reproduces the neuroepithelial aberrations induced by β-catenin. Therefore, we conclude that β-catenin controls the cell fate and polarity of the neuroblasts through the expression and localization of aPKC. Before neurogenesis, the neural tube wall consists of only one cell type, the neuroblasts, from which all neurons and glial cells derive. Neuroepithelial cells form a single-cell-layered pseudostratified epithelium that extends from the apical (ventricular) to the basal lamina and show the typical features of epithelial cells, notably an apical-to-basal polarity. Neuroblasts initially proliferate in a symmetric (self-expanding) mode in order to increase the number of progenitors. With the onset of neurogenesis, asymmetric (self-replacing) divisions give rise to one progenitor and a committed neuron in each round [1] . The proteins present at the apical pole of neuroblasts, collectively called apical complex (AC), are distributed into three concentric sub-domains, where fate-determining factors (par3, atypical protein kinase C (aPKC)) are confined within or close to the apical membrane, zonular proteins (ZO-1, Afadin) occupy an intermediary position and the junctional complexes (N-cadherin, α-catenin and β-catenin) are located at the sub-apical domain [2] . While the distribution during cell division of fate-determining factors is important in determining the fate of the daughter cells [1] , the adherens junctions (AJs) promote the attachment of the neuroblasts within the epithelium and favour the recruitment and stability of the AC components [3] . Although the mechanisms controlling the mode of division are still unclear, it is believed that symmetric divisions occur with a division plane nearly perpendicular to the epithelium, whereas divisions along other planes are asymmetric. As a consequence, although the AJ is always inherited by both daughter cells, the fate determinants may be inherited disproportionately [2] , [4] , [5] . β-Catenin mediates the canonical Wnt pathway through stimulating Tcf-dependent transcription [6] , [7] . However, β-catenin also has pivotal roles in epithelial cell polarity, and by associating with classic cadherins via its armadillo domains it contributes to their membrane delivery [3] . Moreover, through α-catenin, β-catenin links AJ to the apical actin belt [8] . Accordingly, it remains unclear whether the role of β-catenin in cell polarity and epithelium integrity is due to its transcriptional activity, its structural role or both. Here we have used an in vivo model to study the contribution of β-catenin on polarity maintenance and fate acquisition along neuroepithelium development that involves the electroporation of a stable form of β-catenin (sβ-catenin) into the neuroepithelial cells of the chick embryo neural tube. Taking advantage of this in vivo model, we found that sustained activity of β-catenin maintains the stemness of neuroblasts and it inhibits their differentiation, causing aberrant growth in the neuroepithelium. Thus, we used this model to explore the transcriptional and structural roles of β-catenin during the initiation of malformations. We show that β-catenin/Tcf transcriptional activity is required for the expression of aPKC, a necessary AC component. Additionally, we show that a non-transcriptional role of β-catenin is required to drive the sub-cellular distribution of aPKC and its activation in the apical pole of neuroepithelial cells. Finally, we demonstrate that β-catenin-induced neuroepithelial aberrations can be reproduced by constitutively active forms of aPKC, and prevented by ‘kinase-dead’ aPKC mutants with dominant negative activity. We conclude that while β-catenin activity is required for proper cell polarity and fate acquisition during normal neural tube development, its sustained activation leads to improper aPKC activation at the apical pole of neuroblasts causing severe aberrant growth of the neuroepithelium. sβ-Catenin causes aberrant growth of neuroepithelium Germline mutations in the WNT inhibitor APC and somatic mutations of the effector of the Wnt pathway CTNNB1 , the gene encoding β-catenin [9] , [10] may cause medulloblastoma, a central nervous system malignancy. Notably, the majority of mutations that activate the Wnt pathway target residues 33–37 of β-catenin, the GSK-3β phosphorylation domain [11] , [12] , rendering meta-stable forms of β-catenin (sβ-catenin). To study the effect of sustained β-catenin activation along neural tube development, here we used the PiggyBac system [13] to permanently express sβ-catenin in the chick embryo hindbrain ( Fig. 1a ). 4′,6-diamidino-2-phenylindole and hematoxylin and eosin staining of the brainstem 7 days post electroporation revealed diverse cytological abnormalities, including the protrusion of tissue masses into the IV ventricle, epithelial discontinuities and ectopic epithelial formations deep into the neural tissue ( Fig. 1b arrows, Supplementary Fig. 1 ). Immunohistochemistry (IHC) for green fluorescent protein (GFP) and for the proliferation marker, proliferating cell nuclear antigen (PCNA), revealed that these masses contained cells expressing sβ-catenin, a fraction of which were proliferating ( Fig. 1c ). Additionally, the distribution of the pan-progenitor marker Sox2, which labels all neuroepithelial cells, confirmed that the neuroepithelial structure was severely disrupted and that the ectopic lumens were surrounded by cells expressing Sox2 ( Fig. 1d arrows). Moreover, at 15 days post electroporation of sβ-catenin, the cell masses filled the IV ventricle ( Fig. 1e ); however, none of the sβ-catenin+ masses adhered to or invaded the cerebellum (labelled with Pax6) at this stage ( Fig. 1e ). Notably, we found that only a fraction of the sβ-catenin+ cells forming the masses were proliferating ( Fig. 1b , Supplementary Fig. 1 ). Thus, we analysed whether an imbalance in the proliferation/differentiation equilibrium underlies the formation of these masses. We analysed the expression of the pan-progenitor marker Sox2 and the pan-neural marker NeuroD as reporters, and 24/48 h post electroporation (h.p.e.) of sβ-catenin, we detected a significant reduction in NeuroD expression that was concomitant with an increase in Sox2 expression ( Fig. 2a ). Notably, 48 h.p.e., sβ-catenin+ cells expressed Sox2 and were retained within the ventricular zone (VZ), causing neuroepithelial aberrations all along the neuraxis including invaginations and extra-lumen formation (spinal cord Fig. 2b left, hindbrain Supplementary Fig. 2 ). Moreover, lateral migration of sβ-catenin+ cells into the mantle zone was impaired, as was the expression of the pan-neural marker HuCD ( Fig. 2b right, quantitative data in Supplementary Fig. 3 ). The epithelial aberrations caused by sβ-catenin 48 h.p.e. were very similar at the different rostro-caudal levels studied, suggesting the disruption of a basic cellular mechanism implicated in neuroepithelium integrity ( Supplementary Fig. 2 ). 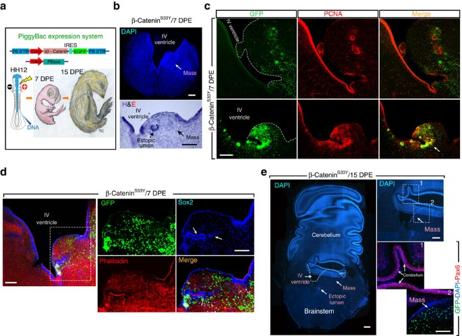Figure 1: Electroporation of a stable form of β-catenin causes aberrant growth of the neuroepithelium. (a) HH-12 chicken embryos were electroporated with β-cateninS33Yin PiggyBac expression system vectors and left to develop for 7 or 15 days post electroporation (DPE). (b) 4′,6-diamidino-2-phenylindole (DAPI) and hematoxylin and eosin (H&E) staining of transverse brainstem sections at 7 DPE; scale bar, 150 μm. (c) Higher-magnification images of brainstem sections showing two examples of the aberrant accumulation of cells stained with antibodies against GFP (green, transfection) and proliferating cell nuclear antigen (PCNA) (red, mitosis marker). (d) Similar sections as incwere stained with phalloidin (red, labels F-actin) and antibodies against GFP (green, transfection) and Sox2 (blue, progenitor marker). (e) DAPI staining of 15 DPE transverse brainstem sections in which the floor of the IV ventricle and the mass are bounded by a dotted line. The right lower panels show amplifications of the two areas indicated by dotted squares in the upper panel that are labelled 1 and 2. Sections were stained with DAPI (blue) and antibodies against GFP (green, transfection) and Pax6 (red, marker of the external germinative layer of the cerebellum). Scale bar, 150 μm. Figure 1: Electroporation of a stable form of β-catenin causes aberrant growth of the neuroepithelium. ( a ) HH-12 chicken embryos were electroporated with β-catenin S33Y in PiggyBac expression system vectors and left to develop for 7 or 15 days post electroporation (DPE). ( b ) 4′,6-diamidino-2-phenylindole (DAPI) and hematoxylin and eosin (H&E) staining of transverse brainstem sections at 7 DPE; scale bar, 150 μm. ( c ) Higher-magnification images of brainstem sections showing two examples of the aberrant accumulation of cells stained with antibodies against GFP (green, transfection) and proliferating cell nuclear antigen (PCNA) (red, mitosis marker). ( d ) Similar sections as in c were stained with phalloidin (red, labels F-actin) and antibodies against GFP (green, transfection) and Sox2 (blue, progenitor marker). ( e ) DAPI staining of 15 DPE transverse brainstem sections in which the floor of the IV ventricle and the mass are bounded by a dotted line. The right lower panels show amplifications of the two areas indicated by dotted squares in the upper panel that are labelled 1 and 2. Sections were stained with DAPI (blue) and antibodies against GFP (green, transfection) and Pax6 (red, marker of the external germinative layer of the cerebellum). Scale bar, 150 μm. 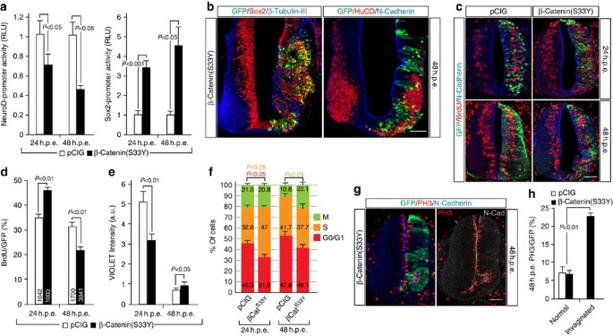Figure 2: sβ-Catenin maintains the stemness of neuroblasts but reduces their proliferation. (a) β-CateninS33Yor the control vector (pCIG) was electroporated along with reporter vectors expressing luciferase driven by the NeuroD or Sox2 promoters. Luciferase activity was assayed at 24 or 48 h.p.e. (b) Transverse sections of HH-12 chicken neural tubes 48 h after electroporation with β-cateninS33Yand stained with antibodies against GFP (green), Sox2 (red) and β-tubulin III (blue, neural differentiation marker) (left panel) or stained for GFP (green, transfection), HuCD (red, neural differentiation marker) and N-cadherin (blue, adherens junction marker) (right panel). (c,d) Representative images and cell quantification of chicken neural tubes 24 or 48 h after electroporation with β-cateninS33Yor the control vector (pCIG), and stained with antibodies against GFP (green, transfection), BrdU (red, proliferation marker) and N-cadherin (Blue). The total number of GFP+ cells counted at each data point is shown within each bar. (e) Similar experimental conditions as incwere used to perform a violet dilution assay (see Methods for details) and the bar graph shows the mean violet intensity per cell measured by FACS. (f) The cell cycle progression of GFP+ cells was analysed by FACS in HH-12 neural tubes 24 or 48 h after transfection with control (pCIG) or β-cateninS33Y: a minimum of 2,500 GFP+ cells per data point were analysed. (g,h) Representative images and cell quantification of chicken neural tubes 48 h after transfection with the control (pCIG) or β-cateninS33Yvector that were stained against GFP (green, transfection), PH3 (red, M phase marker) and N-cadherin (blue). The percentage of PH3+-transfected cells was evaluated, comparing normal and invaginated portions of the epithelium. The bar graphs show the mean±s.d. of at least three experiments. Significant differences were tested by one-way analysis of vaiance (ANOVA) followed by the Tukey’s test. Scale bar, 50 μm. Full size image Figure 2: sβ-Catenin maintains the stemness of neuroblasts but reduces their proliferation. ( a ) β-Catenin S33Y or the control vector (pCIG) was electroporated along with reporter vectors expressing luciferase driven by the NeuroD or Sox2 promoters. Luciferase activity was assayed at 24 or 48 h.p.e. ( b ) Transverse sections of HH-12 chicken neural tubes 48 h after electroporation with β-catenin S33Y and stained with antibodies against GFP (green), Sox2 (red) and β-tubulin III (blue, neural differentiation marker) (left panel) or stained for GFP (green, transfection), HuCD (red, neural differentiation marker) and N-cadherin (blue, adherens junction marker) (right panel). ( c , d ) Representative images and cell quantification of chicken neural tubes 24 or 48 h after electroporation with β-catenin S33Y or the control vector (pCIG), and stained with antibodies against GFP (green, transfection), BrdU (red, proliferation marker) and N-cadherin (Blue). The total number of GFP+ cells counted at each data point is shown within each bar. ( e ) Similar experimental conditions as in c were used to perform a violet dilution assay (see Methods for details) and the bar graph shows the mean violet intensity per cell measured by FACS. ( f ) The cell cycle progression of GFP+ cells was analysed by FACS in HH-12 neural tubes 24 or 48 h after transfection with control (pCIG) or β-catenin S33Y : a minimum of 2,500 GFP+ cells per data point were analysed. ( g , h ) Representative images and cell quantification of chicken neural tubes 48 h after transfection with the control (pCIG) or β-catenin S33Y vector that were stained against GFP (green, transfection), PH3 (red, M phase marker) and N-cadherin (blue). The percentage of PH3+-transfected cells was evaluated, comparing normal and invaginated portions of the epithelium. The bar graphs show the mean±s.d. of at least three experiments. Significant differences were tested by one-way analysis of vaiance (ANOVA) followed by the Tukey’s test. Scale bar, 50 μm. Full size image Since neural progenitor identity and cell cycle maintenance are tightly linked, we asked whether sβ-catenin overexpression affected the rate of neural progenitor division. Interestingly, the incorporation of bromodeoxyuridine (BrdU) had increased 24 h.p.e. of sβ-catenin, although it had subsequently declined by 48 h.p.e. ( Fig. 2c,d ). Thus, we evaluated the average number of divisions that electroporated cells underwent in vivo using CellTrace Violet, a cytoplasmic retention dye that is diluted upon cell division [14] . Compared with control embryos, the mean CellTrace Violet intensity had decreased at 24 h.p.e. with sβ-catenin, while by 48 h.p.e. it had increased, indicating that neural progenitors overexpressing sβ-catenin initially underwent more divisions but that by 48 h.p.e., their rate of cell division was slower ( Fig. 2e ). To gain further insight into the cell cycle kinetics of sβ-catenin+ cells, we analysed the DNA content by flow cytometry (fluorescence-associated cell sorting (FACS)). While a higher proportion of these cells were in S phase at 24 h.p.e., this was not the case at 48 h.p.e., at which stage the proportion of the sβ-catenin+ cells retained in M phase was significantly higher than in the controls ( Fig. 2f ). Immunostaining with the anti-phosphorylated histone3 (PH3) mitotic marker confirmed the FACS data, further showing that in the areas where the epithelium had invaginated, the percentage of sβ-catenin+ cells arrested in the M phase was higher than in control-transfected embryos or among sβ-catenin+ cells from areas where the epithelium was morphologically normal ( Fig. 2g,h ). Together these results indicated that electroporation of sβ-catenin into the chick embryo neural tube caused an initial acceleration of the cell cycle, as reported previously [15] , which was followed by a deceleration and M phase arrest. Consequently, sβ-catenin+ cells became slow-dividing Sox2+ neural progenitors that were retained within the VZ, where their lateral migration and neurogenesis were impaired. On the other hand, overexpression of MYCN and CCND1 , two direct targets of the Wnt pathway, strongly induces neuroblast proliferation [15] but not epithelial aberrations ( Supplementary Fig. 4 ), demonstrating that the aberrant growth induced by sβ-catenin is not simply caused by the overgrowth of the epithelium. Aberrant growth is caused by apico-basal shrinkage To decipher the cellular processes that provoke the formation of tumour-like cell masses, we first assessed the conservation of this β-catenin activity along the rostral-caudal axis of the developing nervous system. This was achieved by electroporating three different sβ-catenin molecules (β-catenin S37A , β-catenin Δ29–48 and β-catenin S33Y ) into the rhombencephalon or spinal cord ( Fig. 3a ), each of which produced similar malformations evident through Phalloidin staining: profound invaginations of the luminal face of the neuroepithelium with a minor distortion of the basal membrane ( Fig. 3b–e ). The invaginations formed similarly in both rostro-caudal regions, the spinal cord ( Fig. 3c–e ) and rhombencephalon ( Fig. 3b and Supplementary Fig. 2 ). 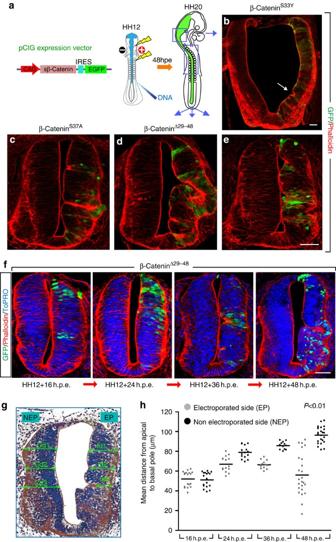Figure 3: Apico-basal shrinkage of sβ-catenin-expressing cells leads to severe malformations of the neuroepithelium. (a–e) HH-12 chicken neural tubes were electroporated with three different stable forms of β-catenin (β-cateninS37A, β-cateninΔ29–48and β-cateninS33Y) at the level of the rhombencephalon (b) and the spinal cord (c–e). Transverse sections were stained with antibodies against GFP (green, transfection) and phalloidin (red, labels F-actin). The arrow inbindicates the invaginated epithelium, note the lower magnification in this panel. (f–h) Chicken embryos were analysed 16, 24, 36 or 48 h after electroporation with β-cateninΔ29–48and transverse sections were stained with antibodies against GFP (green, transfection) and phalloidin (red). Panelgshows a scheme of how the apico-basal distance was measured in the cells forming invaginations. For each Id (invagination distance) measured on the electroporated side (EP), a Cd (control distance) was measured at the same dorso–ventral level on the non-electroporated side (NEP). Panelhshows a dot chart of apical-basal distances at different times after transfection. Scale bar, 50 μm. Figure 3: Apico-basal shrinkage of sβ-catenin-expressing cells leads to severe malformations of the neuroepithelium. ( a – e ) HH-12 chicken neural tubes were electroporated with three different stable forms of β-catenin (β-catenin S37A , β-catenin Δ29–48 and β-catenin S33Y ) at the level of the rhombencephalon ( b ) and the spinal cord ( c – e ). Transverse sections were stained with antibodies against GFP (green, transfection) and phalloidin (red, labels F-actin). The arrow in b indicates the invaginated epithelium, note the lower magnification in this panel. ( f – h ) Chicken embryos were analysed 16, 24, 36 or 48 h after electroporation with β-cateninΔ 29–48 and transverse sections were stained with antibodies against GFP (green, transfection) and phalloidin (red). Panel g shows a scheme of how the apico-basal distance was measured in the cells forming invaginations. For each Id (invagination distance) measured on the electroporated side (EP), a Cd (control distance) was measured at the same dorso–ventral level on the non-electroporated side (NEP). Panel h shows a dot chart of apical-basal distances at different times after transfection. Scale bar, 50 μm. Full size image Analysing the time course of these changes, the first invaginations were evident between 16 and 24 h.p.e., and they were clearly visible at 36 and 48 h.p.e. ( Fig. 3f ). To study the mechanics of invagination, we measured the apico-basal width of the neural tube in the middle of the invagination (Id) and that of the contralateral non-electroporated side at the same dorso–ventral level (Cd: Fig. 3g ). It is worth noting that at this stage, all neuroblasts expand from the apical-to-basal face of the neural tube. When plotted ( Fig. 3h ), it is clear that the width of the neural tube on the non-electroporated side nearly doubled between 16 and 48 h.p.e. due to the appearance of newly generated neurons, and where the sβ-catenin+ cells formed invaginations this distance increased much less. Notably, the apico-basal distance of some regions of the neural tube where invaginations formed was even shorter at 48 h.p.e. than at 16 h.p.e., reflecting the active apico-basal constriction of the cells forming them. Electroporation of empty vector had no effect on neural tube width ( Supplementary Fig. 5 ). These analyses suggest that the migration of sβ-catenin+ cells is impaired, pointing to a structural role of sβ-catenin in the initial formation of the masses. However, since we observed changes in the rate of cell division and the length of the cell cycle, which suggested a transcriptional response, we set out to distinguish between the transcriptional and structural roles of β-catenin at the onset of neuroepithelial malformations. sβ-Catenin effects require Tcf-dependent transcription β-Catenin fulfils dual conserved activities in function of its sub-cellular distribution: in the cytoplasm it binds to cadherins and α-catenin, which in turn associates with F-actin-binding proteins, linking AJs to the actin cytoskeleton [3] , [16] ; in the nucleus it associates with the Tcf transcription factor stimulating the canonical Wnt pathway [6] , [7] . To examine the influence of each of these activities independently, we generated a β-catenin S33Y ΔαCatBs mutant lacking the α-catenin-binding domain [17] ( Supplementary Fig. 6 ), and a truncated β-catenin S33Y ΔCT mutant lacking the last 108 amino acids, which has only very weak transcriptional activity [18] ( Fig. 4a ). In addition, we used three constructs containing the HMG box of the Tcf3 transcription factor: the Tcf3-HMG Box alone that neutralizes Tcf-dependent transcription (Tcf3·HMGB); the HMG box fused to the transactivator domain of VP16 (VP16·Tcf3); or that fused to the repressor domain of the Engrailed protein (EnR·Tcf3: Fig. 4a ). To assess Wnt-dependent transcriptional responses at the cellular level, we generated a 5 × Tcf-bs-RFP (TopRed) reporter (based on the classical 5 × Tcf-bs-Luc, TopFlash). The relative capacity of sβ-catenin and VP16·Tcf3 to stimulate Tcf-dependent transcription was studied in neuroepithelial cells electroporated with TopFlash and the responsiveness of TopRed reporter was tested by transfecting EnR·Tcf3 or VP16·Tcf3 into human embryonic kidney cells (HEK) ( Fig. 4a ). Co-electroporation of TopRed with the control pCIG/GFP vector labelled the endogenous Wnt-responding domain in the dorsal neural tube ( Fig. 4b ), demonstrating that TopRed is a bona fide reporter of Wnt activity. 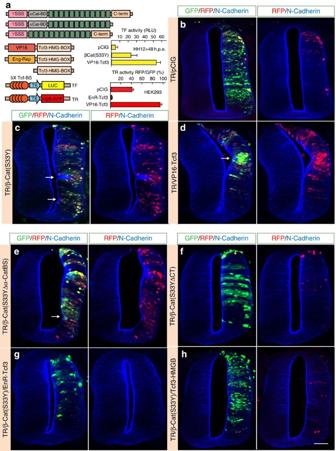Figure 4: sβ-Catenin requires Tcf-dependent transcription but not binding to α-catenin to induce neuroepithelial malformations. (a) Scheme of the different DNA constructs used in the figure, all constructs except the reporters (TopFlash and TopRed), were cloned into pCIG. Modulators of Tcf-dependent transcription contained a Tcf3-HMG box alone (Tcf3-HMGB) or that was fused to the VP16 activator (VP16-Tcf3) or the Engrailed repressor (EnR-Tcf3). TopFlash and TopRed reporter constructs contained a 5 × Tcf-binding motive controlling luciferase and RFP, respectively. The transcriptional strength of β-cateninS33Yand Vp16·Tcf3 was compared with TopFlash in HH-12 chicken embryos. The performance of TopRed was assessed in human embryonic kidney-293 with VP16·Tcf3 and EnR·Tcf3. (b–h) The different construct combinations were analysed 48 h after electroporation into HH-12 chicken neural tubes. Transverse sections were stained with antibodies against GFP (green, transfection), RFP (red, Tcf-dependent activity) and N-cadherin (blue). The green channel has been omitted in the picture at the right of each panel for clarity. Arrows indicate the invaginations. The absence of α-catenin binding by the mutant used in panele(β-cateninS33YΔαCatBs) is shown inSupplementary Fig. 6. Scale bar, 50 μm. Figure 4: sβ-Catenin requires Tcf-dependent transcription but not binding to α-catenin to induce neuroepithelial malformations. ( a ) Scheme of the different DNA constructs used in the figure, all constructs except the reporters (TopFlash and TopRed), were cloned into pCIG. Modulators of Tcf-dependent transcription contained a Tcf3-HMG box alone (Tcf3-HMGB) or that was fused to the VP16 activator (VP16-Tcf3) or the Engrailed repressor (EnR-Tcf3). TopFlash and TopRed reporter constructs contained a 5 × Tcf-binding motive controlling luciferase and RFP, respectively. The transcriptional strength of β-catenin S33Y and Vp16·Tcf3 was compared with TopFlash in HH-12 chicken embryos. The performance of TopRed was assessed in human embryonic kidney-293 with VP16·Tcf3 and EnR·Tcf3. ( b – h ) The different construct combinations were analysed 48 h after electroporation into HH-12 chicken neural tubes. Transverse sections were stained with antibodies against GFP (green, transfection), RFP (red, Tcf-dependent activity) and N-cadherin (blue). The green channel has been omitted in the picture at the right of each panel for clarity. Arrows indicate the invaginations. The absence of α-catenin binding by the mutant used in panel e (β-catenin S33Y ΔαCatBs) is shown in Supplementary Fig. 6 . Scale bar, 50 μm. Full size image Co-electroporation of β-catenin S33Y with TopRed showed that the neuroepithelial malformations contained transfected cells and expressed high levels of red fluorescent protein (RFP) ( Fig. 4c ). However, similar levels of RFP were evident with VP16·Tcf3 even though small invaginations were generated ( Fig. 4d ). β-Catenin S33Y ΔαCatBs, which did not bind to α-catenin, induced a similar cellular and transcriptional response to β-catenin S33Y ( Fig. 4e ), while β-catenin S33Y ΔCT that has no transcriptional activity formed no invaginations and displayed similar RFP expression to the controls, in the endogenous Wnt domain alone ( Fig. 4f ). In addition, we found that β-catenin S33Y -induced malformations and RFP expression were both totally reverted by the co-expression of Tcf3·HMGB or EnR·Tcf3 ( Fig. 4g,h ). Together these experiments demonstrated that the β-catenin to α-catenin association was not required for the retention of β-catenin+ cells within the VZ and for the formation of neuroepithelial malformations. By contrast, the transcriptional activity of β-catenin appeared to be absolutely necessary for the neuroepithelial malformations, prompting us to search for the putative targets of this transcriptional activity that might prevent the delamination and differentiation of β-catenin+ cells. β-Catenin regulates the formation of the AC Primary neurogenesis is initiated by the onset of asymmetric divisions that generate a stem cell daughter that remains as a progenitor within the VZ and another daughter cell committed to differentiation that migrates laterally towards the marginal zone. Neural progenitors within the VZ retain an apico-basal polarity where ACs are found at the luminal face. The role played by the AC in the maintenance of neural stem cell identity is only just beginning to be understood [2] , [4] , [5] and thus, we set to analyse whether the overexpression of stable β-catenin affects components of the AC. There was a significant increase in the total amount of N-cadherin and aPKC detected in western blots (WBs) of extracts from neural tubes transfected with sβ-catenin, while other components of the AC were not significantly altered, such as ZO-1 ( Fig. 5a ). Hence, the expression of some but not all components of the AC appears to be regulated by β-catenin activity. We investigated the sub-cellular distribution of these components of the AC and dual immunostaining showed that electroporated sβ-catenin mainly co-localized with N-cadherin at the apical pole ( Fig. 5b ). Moreover, in isolated sβ-catenin+ cells ZO-1 ( Fig. 5c ), aPKC ( Fig. 5d ) and N-cadherin ( Fig. 5c,d ) were all localized to the apical pole, and when quantified, there was significantly more endogenous N-cadherin and aPKC in sβ-catenin+ cells than in non-electroporated cells, especially in the cells forming invaginations ( Fig. 5e : see methods for the details of quantification). Furthermore, the P-aPKC/aPKC (active/inactive) ratio was clearly higher at the invaginations generated by sβ-catenin+ expression ( Fig. 5f ). Together these experiments indicate that β-catenin activity was sufficient to not only increase the expression of AC components but also to drive their localization to the apical pole, notably N-cadherin and aPKC. On the other hand, direct overexpression of N-cadherin or the expression of molecules that increased either N-cadherin recruitment (PAR3) or stability (p120 CNT ) failed to induce invaginations ( Supplementary Fig. 7 ). Next, we assessed whether the oversized ACs appeared at the time of sβ-catenin-induced epithelial abnormalities ( Fig. 5g ) and we found that cells with enlarged ACs appeared normal at interphase ( Fig. 5g , interphase). However, the β-catenin+ cells underwent mitosis deeper in the epithelium than non-transfected cells ( Fig. 5g , compare arrow and arrowhead in early mitosis panel), causing small invaginations of the luminal face ( Fig. 5g late mitosis) and suggesting a malfunction of spindle orientation and/or of the forces driving cytokinesis, phenomena that could explain the M phase arrest caused by sβ-catenin (shown in Fig. 2 ). Thus, we examined whether Tcf was required for normal AC formation and function by co-electroporating two potent transcriptional repressors to completely abolish Tcf-mediated transcription: the EnR·Tcf3 together with a dominant negative form of Tcf4 (ref. 15 ) (DNTcf4: Fig. 5h ). The loss of Tcf function resulted in a cell autonomous loss of N-cadherin and aPKC expression ( Fig. 5h arrowheads), and a mislocalization of ZO-1 ( Fig. 5i ) at the apical pole. Notably, some of these cells that lacked an AC were found in the ventricle forming agglomerations of round unpolarized cells ( Fig. 5h , arrowhead in enlarged lower panel). Together these data showed that Tcf activity is required for the formation of the AC, prompting us to study whether Tcf activity was sufficient for the formation of the AC. 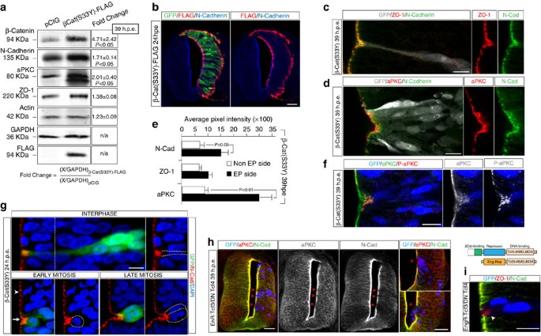Figure 5: β-Catenin regulates AC formation. Electroporations were performed in HH-12 chicken embryos. Scale bars represent 10 μm inc,d,f,g,iand 50 μm inb–h. (a) Neural tubes were electroporated with control (pCIG) or β-cateninS33Yand AC proteins assessed by WB. Protein levels were normalized to the glyceraldehyde 3-phosphate dehydrogenase (GAPDH), and the difference between control and β-cateninS33Ywas calculated. Fold change=mean of three experiments ±s.d. (b) Neural tubes were electroporated with β-cateninS33Y·FLAG and stained with antibodies against GFP (green, transfection), FLAG (red, β-cateninS33Ydistribution) and N-cadherin (blue). (c–e) Representative high-magnification images and pixel intensity quantification (see Methods for statistics) of neural tubes transfected with β-cateninS33Yand stained against GFP (greys, transfection), ZO-1 (red inc) or aPKC (red ind) and N-cadherin (green). (f) Similar sections to those incwere stained against GFP (blue, transfection), aPKC (green) and P-aPKC (red). The separate channels are shown in grey for comparison. (g) Neural tubes were electroporated with β-cateninS33Yand stained against GFP (green, transfection), N-cadherin (red) and 4′,6-diamidino-2-phenylindole (DAPI) (blue, labels DNA). The three panels show β-cateninS33Y+ cells at three different stages of the cell cycle. In the early mitosis panel, two cells with condensed chromosomes are indicated (arrowhead=non-transfected, arrow=β-cateninS33Y+). An image omitting the GFP channel is shown to the right of each panel for clarity. (h) Neural tubes were electroporated with Eng·Tcf3 plus a dominant negative Tcf4 (DN Tcf4, a scheme of the constructs is shown to the right of the pictures), sections were stained against GFP (blue, transfection), aPKC (red) and N-caderin (green). Arrowheads point to discontinuities in the ACs coincident with transfected cells. Two enlarged images showing areas of transfected cells with AC deficiencies (arrowheads) are shown at the right of the pannel. (i) Very high-magnification image of a section as inh, ZO-1 is mislocated in cells with no N-cadherin at the AJs (arrowhead). Sections stained with GFP (blue, transfection), ZO-1 (red) and N-cadherin (green). Figure 5: β-Catenin regulates AC formation. Electroporations were performed in HH-12 chicken embryos. Scale bars represent 10 μm in c , d , f , g , i and 50 μm in b – h . ( a ) Neural tubes were electroporated with control (pCIG) or β-catenin S33Y and AC proteins assessed by WB. Protein levels were normalized to the glyceraldehyde 3-phosphate dehydrogenase (GAPDH), and the difference between control and β-catenin S33Y was calculated. Fold change=mean of three experiments ±s.d. ( b ) Neural tubes were electroporated with β-catenin S33Y ·FLAG and stained with antibodies against GFP (green, transfection), FLAG (red, β-catenin S33Y distribution) and N-cadherin (blue). ( c – e ) Representative high-magnification images and pixel intensity quantification (see Methods for statistics) of neural tubes transfected with β-catenin S33Y and stained against GFP (greys, transfection), ZO-1 (red in c ) or aPKC (red in d ) and N-cadherin (green). ( f ) Similar sections to those in c were stained against GFP (blue, transfection), aPKC (green) and P-aPKC (red). The separate channels are shown in grey for comparison. ( g ) Neural tubes were electroporated with β-catenin S33Y and stained against GFP (green, transfection), N-cadherin (red) and 4′,6-diamidino-2-phenylindole (DAPI) (blue, labels DNA). The three panels show β-catenin S33Y + cells at three different stages of the cell cycle. In the early mitosis panel, two cells with condensed chromosomes are indicated (arrowhead=non-transfected, arrow=β-catenin S33Y +). An image omitting the GFP channel is shown to the right of each panel for clarity. ( h ) Neural tubes were electroporated with Eng·Tcf3 plus a dominant negative Tcf4 (DN Tcf4, a scheme of the constructs is shown to the right of the pictures), sections were stained against GFP (blue, transfection), aPKC (red) and N-caderin (green). Arrowheads point to discontinuities in the ACs coincident with transfected cells. Two enlarged images showing areas of transfected cells with AC deficiencies (arrowheads) are shown at the right of the pannel. ( i ) Very high-magnification image of a section as in h , ZO-1 is mislocated in cells with no N-cadherin at the AJs (arrowhead). Sections stained with GFP (blue, transfection), ZO-1 (red) and N-cadherin (green). Full size image Accordingly, we took advantage of the VP16·Tcf3 construct, which is capable of stimulating Tcf-dependent transcription in the absence of β-catenin [19] . Electroporation of VP16·Tcf3 alone resulted in smaller neuroepithelial invaginations than the malformations caused by the electroporation of sβ-catenin alone ( Fig. 6a ), even though this construct was capable of intensely activating the Wnt pathway ( Fig. 4d ). When we assessed the expression of AC components, we found that VP16-Tcf3+ cells strongly expressed aPKC, an effect that was cell autonomous ( Fig. 6b ). Moreover, the excess aPKC protein was distributed throughout the cytoplasm and it was not restricted to the AC ( Fig. 6b arrow). The expression of N-cadherin, β-catenin or ZO-1 was not influenced by VP16·Tcf3 electroporation ( Fig. 6b ) and notably, we observed groups of round unpolarized Vp16·Tcf3+ cells at the lumen ( Fig. 6b , arrowheads). Interestingly, although both sβ-catenin and VP16·Tcf3 electroporation resulted in comparable quantitative induction of aPKC mRNA expression (aPKCζ and ı mRNA levels measured by reverse transcriptase real-time PCR) ( Fig. 6c ), the cellular response was qualitatively quite different. While VP16-Tcf3+ cells accumulate aPKC in the cytoplasm ( Fig. 6b ), aPKC augmented at the AC in sβ−catenin+ cells ( Fig. 5e,g ), indicating that β-catenin fulfils obligations independent of transcription that contribute to aPKC delivery to the apical pole. When we tested this possibility by co-electroporating sβ-catenin and VP16-Tcf3, the excess aPKC was redistributed to the AC ( Fig. 6d ). Hence, β-catenin appears to control aPKC transcription and localization through Tcf-dependent and -independent mechanisms. 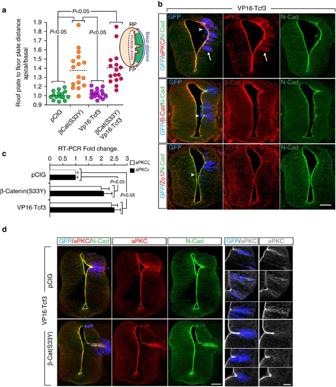Figure 6: β-Catenin regulates the expression and location of aPKC through Tcf-dependent and -independent mechanisms. (a) HH-12 chicken neural tubes were electroporated with control (pCIG), β-cateninS33Y, Vp16·Tcf3 or both and analysed 48 h later. The distance from the roof to the floorplate was measured at the apical (apical distance) and basal (basal distance) faces of the epithelium, and the ratio between them was plotted. For each treatment, four sections from each of four embryos were measured. (b) Vp16·Tcf3-transfected sections were stained after 48 h with antibodies against GFP (blue, transfection), aPKC, β-catenin or ZO-1 (red) and N-cadherin (green). Arrowheads indicate groups of cells in the ventricle and the arrows Vp16·Tcf3+ cells with cytoplasmic accumulations of aPKC. (c) The aPKCı and aPKCζ mRNAs were measured by real-time PCR in chicken neural tubes 48 h after transfection with control (pCIG), β-cateninS33Yor Vp16·Tcf3, five embryos per data point were pooled. The bar graphs show the mean±s.d. of three experiments. Significant differences were tested by one-way analysis of variance (ANOVA) followed by the Tukey’s test. (d) Chicken neural tubes were stained with antibodies against GFP (blue, transfection), aPKC (red) and N-cadherin (green) 48 h after electroporation with Vp16·Tcf3 or Vp16·Tcf3 plus β-cateninS33Y. The right panel shows enlarged images of three more examples of the effect of control or β-cateninS33Yexpression on the distribution of aPKC, these pictures are displayed in grey scale for better comparison. Scale bar represents 50 μm inb,d(left) and 25 μm ind(right). Figure 6: β-Catenin regulates the expression and location of aPKC through Tcf-dependent and -independent mechanisms. ( a ) HH-12 chicken neural tubes were electroporated with control (pCIG), β-catenin S33Y , Vp16·Tcf3 or both and analysed 48 h later. The distance from the roof to the floorplate was measured at the apical (apical distance) and basal (basal distance) faces of the epithelium, and the ratio between them was plotted. For each treatment, four sections from each of four embryos were measured. ( b ) Vp16·Tcf3-transfected sections were stained after 48 h with antibodies against GFP (blue, transfection), aPKC, β-catenin or ZO-1 (red) and N-cadherin (green). Arrowheads indicate groups of cells in the ventricle and the arrows Vp16·Tcf3+ cells with cytoplasmic accumulations of aPKC. ( c ) The aPKCı and aPKCζ mRNAs were measured by real-time PCR in chicken neural tubes 48 h after transfection with control (pCIG), β-catenin S33Y or Vp16·Tcf3, five embryos per data point were pooled. The bar graphs show the mean±s.d. of three experiments. Significant differences were tested by one-way analysis of variance (ANOVA) followed by the Tukey’s test. ( d ) Chicken neural tubes were stained with antibodies against GFP (blue, transfection), aPKC (red) and N-cadherin (green) 48 h after electroporation with Vp16·Tcf3 or Vp16·Tcf3 plus β-catenin S33Y . The right panel shows enlarged images of three more examples of the effect of control or β-catenin S33Y expression on the distribution of aPKC, these pictures are displayed in grey scale for better comparison. Scale bar represents 50 μm in b , d (left) and 25 μm in d (right). Full size image Aberrant growth is mediated by aPKCı The binding of aPKC to Par6 drives its folding into a low-activity conformation, whereby the kinase domain at the C terminus of aPKC binds to a pseudo-substrate motive at the N terminus. Par3 directs the aPKC–Par6 complex to the apical pole, where Cdc42 activity disrupts the association of aPCK with Par6, and PDK1 phosphorylates aPKC at T403–410 to fully activate it [20] , [21] . Having demonstrated a role for β-catenin/Tcf in the expression, sub-cellular localization and activation of aPKC at the AC of neuroepithelial cells, we assessed whether aPKC alone was sufficient to mimic the role of sβ-catenin in driving pre-neoplastic growth in the neuroepithelium. Unlike wild-type aPKCζ, expression of aPKCζ ΔNT , a constitutively active N-terminus-deleted aPKC mutant that does not bind to Par6, induced the delamination of neuroepithelial cells [22] . Similarly, we observed no phenotypic changes following aPKCζ·GFP transfection, yet electroporation of aPKCζ ΔNT induced a cell autonomous, ectopic accumulation of AC proteins at 16 h.p.e. (N-cadherin, ZO-1 and F-actin: Fig. 7a and arrowheads in Fig. 7b ), as well as neuroepithelial malformations resembling those induced by sβ-catenin (spinal cord Fig. 7b , hindbrain Supplementary Fig. 8 ). Moreover, similarly to sβ-catenin, aPKCζ ΔNT -expressing cells remained as Sox2+ progenitors and did not differentiate ( Supplementary Fig. 9 ). Indeed, aPKCζ ΔNT totally disrupted the polarity of the neuroepithelium at 39 h.p.e., as well as the distribution of the accumulated AC proteins in transfected cells ( Fig. 7b ). We have shown that the cytoplasmic accumulation of aPKC induced by VP16·Tcf3 was redistributed to the AC by sβ-catenin ( Fig. 5d ). Similarly, the cytoplasmic accumulation of overexpressed wild-type aPKCı was restricted to the apical pole in the neuroepithelial cells co-expressing sβ-catenin ( Fig. 7c ). In addition, sβ-catenin redirected aPKCζ ΔNT to the apical pole and more importantly, it prevented the depolarization caused by this constitutively active mutant. In fact, the lesions observed in aPKCζ ΔNT plus sβ-catenin were indistinguishable from those in sβ-catenin alone ( Fig. 7d ), strongly suggesting that the accumulation of active aPKC at the AC was the main driver of sβ-catenin-induced malformations. To confirm this hypothesis, we studied the effect of suppressing aPKC. 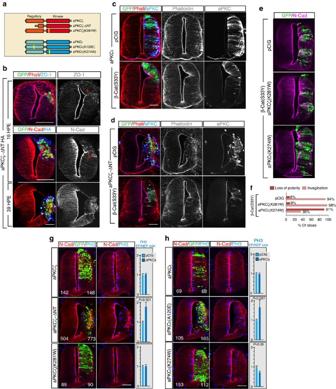Figure 7: β-Catenin activation of aPKCı is both necessary and sufficient for the pre-neoplastic malformations of the neuroepithelium. (a) Scheme of the DNA constructs used in the figure. (b) HH-12 chicken neural tubes were analysed 16 (two upper panels) or 39 h (lower panel) after electroporation with aPKCζΔNT·HA. Sections were stained with antibodies against GFP (green, transfection), phalloidin (labels F-actin) or N-cadherin (red) and ZO-1or HA (blue). Arrowheads indicate ectopic accumulation of ZO-1 and N-cadherin. (c) Neural tubes were stained with phalloidin (red), and with antibodies against GFP (green, transfection) and aPKC (blue) 39 h after electroporation with aPKCı alone or plus β-cateninS33Y. Isolated channels are shown in grey scale for a better comparison. (d) Similar experimental conditions as incbut following transfection of aPKCζΔNT. (e) Chicken neural tubes 39 h after transfection with β-cateninS33Yplus pCIG (control), aPKCζK281Wor aPKCıK274W(kinase-dead mutants). Sections were stained with antibodies against GFP (green, transfection) and N-cadherin (magenta). (f) The bar graph shows the percentage of sections from the experiment shown inethat presented invaginations and/or a loss of polarity for each treatment. The total number of sections studied (n) in each condition was pCIG=48, aPKCıK274W=62, aPKCζK281W=45. (g,h) Sections of chicken neural tubes were stained with antibodies against GFP (green, transfection), N-cadherin (red) and PH3 (blue) 39 h after electroporation with wild type (aPKCζ, and aPKCı), active (aPKCζΔNTand aPKCıA120E) or kinase-dead (aPKCζK281Wand aPKCıK274W) mutants of the ζ and ı isoforms of aPKC. The ratio obtained by dividing the number of PH3+ cells in the electroporated side (EP) by the non-electroporated one (NE) is plotted to the right of each treatment. The number of PH3+ cells counted (n) is displayed within each photogram (white lettering). The bar graphs show the mean±s.d. Significant differences were tested by one-way analysis of variance (ANOVA) followed by the Tukey’s test. Scale bar, 50 μm. Figure 7: β-Catenin activation of aPKCı is both necessary and sufficient for the pre-neoplastic malformations of the neuroepithelium. ( a ) Scheme of the DNA constructs used in the figure. ( b ) HH-12 chicken neural tubes were analysed 16 (two upper panels) or 39 h (lower panel) after electroporation with aPKCζ ΔNT ·HA. Sections were stained with antibodies against GFP (green, transfection), phalloidin (labels F-actin) or N-cadherin (red) and ZO-1or HA (blue). Arrowheads indicate ectopic accumulation of ZO-1 and N-cadherin. ( c ) Neural tubes were stained with phalloidin (red), and with antibodies against GFP (green, transfection) and aPKC (blue) 39 h after electroporation with aPKCı alone or plus β-catenin S33Y . Isolated channels are shown in grey scale for a better comparison. ( d ) Similar experimental conditions as in c but following transfection of aPKCζ ΔNT . ( e ) Chicken neural tubes 39 h after transfection with β-catenin S33Y plus pCIG (control), aPKCζ K281W or aPKCı K274W (kinase-dead mutants). Sections were stained with antibodies against GFP (green, transfection) and N-cadherin (magenta). ( f ) The bar graph shows the percentage of sections from the experiment shown in e that presented invaginations and/or a loss of polarity for each treatment. The total number of sections studied ( n ) in each condition was pCIG=48, aPKCı K274W =62, aPKCζ K281W =45. ( g , h ) Sections of chicken neural tubes were stained with antibodies against GFP (green, transfection), N-cadherin (red) and PH3 (blue) 39 h after electroporation with wild type (aPKCζ, and aPKCı), active (aPKCζ ΔNT and aPKCı A120E ) or kinase-dead (aPKCζ K281W and aPKCı K274W ) mutants of the ζ and ı isoforms of aPKC. The ratio obtained by dividing the number of PH3+ cells in the electroporated side (EP) by the non-electroporated one (NE) is plotted to the right of each treatment. The number of PH3+ cells counted ( n ) is displayed within each photogram (white lettering). The bar graphs show the mean±s.d. Significant differences were tested by one-way analysis of variance (ANOVA) followed by the Tukey’s test. Scale bar, 50 μm. Full size image Both of the active forms of aPKCζ and aPKCı (aPKCζ ΔNT and aPKCı A120E , respectively) initiated sβ-catenin-like invaginations at 16 h.p.e. ( Fig. 7b ), therefore we transfected kinase-‘dead’ (kinase inactive) forms of aPKCζ and aPKCı (aPKCζ K281W and aPKCı K274W , respectively) to assess the individual contribution of each aPKC isoform to the sβ-catenin-induced malformations. Notably, we observed that aPKCı K274W but not aPKCζ K281W significantly decreased the number of tissue malformations ( Fig. 7e,f ). Additionally, in most aPKCı K274W -transfected sections, we observed groups of non-polarized cells with no AC ( Fig. 7e,f ), very much resembling the EnR·Tcf3/DNTcf4-transfected cells seen previously ( Fig. 5h ). Accordingly, we used the constitutively active or kinase-dead mutants of aPKCζ, and aPKCı, in an attempt to fully understand the role played by aPKC isoforms on AC formation, and therefore in sβ-catenin-induced malformations. We electroporated the neural tube with the distinct aPKC constructs and analysed AC protein accumulation (with anti-N-cadherin) and M phase arrest (with anti PH3), two characteristic abnormalities in sβ-catenin lesions. While neither of the wild-type forms produced tissue malformations ( Fig. 7g,h ), both the active forms induced abundant ectopic ACs and a significant increase of cells in M phase, neither of which were restricted to the luminal face but rather occurred at any position in the neuroepithelium ( Fig. 7g,h ). Conversely, striking differences were observed when the effects of the aPKCζ and aPKCı kinase-dead mutants were compared. While aPKCζ K281W provoked no anomalies, aPKCı K274W -expressing cells did not form ACs and were less often found in M phase ( Fig. 7g,h ), strongly supporting a role for the aPKCı isoform in these events. Together our results demonstrated that sβ-catenin induces neuroepithelial lesions involving morphological tissue invaginations, where cells remain as progenitors and are arrested in the M phase of the cell cycle, and where they accumulate an excess of AC proteins. The activity of aPKC is sufficient to reproduce the phenotype, including the arrest at M phase. Indeed, aPKCı activity is not only required for the production of sβ-catenin-induced lesions but also for normal AC formation, which is in turn essential for M phase progression. Neuroblasts are the primary embryonic stem cells in the nervous system that initially proliferate in a symmetric (self-expanding) mode in order to increase the number of progenitors. With the onset of neurogenesis, asymmetric (self-replacing) divisions give rise to one progenitor and a committed neuron in each round. Although the mechanisms controlling the mode of division are still unclear, it is believed that symmetric divisions occur with a division plane nearly perpendicular to the epithelium, whereas divisions along other planes are asymmetric. As a consequence, although the AJ is always inherited by both daughter cells, the fate determinants (aPKC, Par3) may be inherited disproportionately [2] , [4] , [5] . Active forms of aPKC increase the number of Sox2-positive progenitors in the chick neural tube [22] and during Xenopus neurogenesis [23] , cells expressing aPKC ΔNT remain as progenitors and they do not differentiate ( Supplementary Figs 8e and 9 ). Thus, if the apical division model proposed by Marthiens and Ffrench-Constant is applied [5] , enlarged ACs, as observed in sβ-catenin+ cells, would provide sufficient fate determinants to both daughter cells for them to remain as progenitors, regardless of the plane of division. We also found that sβ-catenin causes active aPKC to accumulate at the apical pole through a combination of transcriptional and non-transcriptional mechanisms, and that active aPKC is sufficient to induce the accumulation of N-cadherin. Thus, sβ-catenin and active aPKC induce both, stemness and accumulation of N-cadherin; in agreement, Foxp repression of N-cadherin transcription during neural tube development induces detachment and differentiation of neuroblasts [24] . On the other hand, N-cadherin stability at the plasma membrane is enhanced by its association with P120 ctn through its cytoplasmic domain [25] ; however, it should be noted that the sβ-catenin phenotype was not reproduced by p120 ctn or N-cadherin overexpression ( Supplementary Fig. 7 ). In addition, active aPKC also induced ZO-1 accumulation and therefore, either aPKC activates a mechanism that promotes the stability of the entire AC or, as proposed elsewhere [3] , N-cadherin can recruit the other components of the AC. The tissue malformations induced by sβ-catenin consist of initial neuroepithelium invaginations that end up creating ectopic lumens and rosette-like structures where the epithelial sheets remain mitotically active deep in the neural tissue. In addition, we found that invaginations started during mitosis of the sβ-catenin+ cells, notably the same cells that were arrested in M phase, suggesting that the forces distorting the epithelium and obstructing the normal completion of mitosis could have a common origin. The position and orientation of the mitotic spindle are determined by forces generated at the cell cortex, where astral microtubules emanating from the mitotic spindle pole are anchored to the plasma membrane [26] . However, for several reasons this process could be impaired in cells presenting enlarged ACs. The membrane-anchored Gα–LGN–NuMA complex interacts with the microtubule-associated minus-end motor Lis1-Dynein-Dynactin, generating the traction forces that position the mitotic spindle. Accordingly, LGN is required for planar cell division and to maintain progenitors in the chick neuroepithelium [27] . Astral microtubules interact with the Gα–LGN–NuMA complex located at the basolateral membrane below the AJs, apical anchoring being prevented by apical aPKC through the phosphorylation of LGN [28] and NuMA [29] . In addition, direct binding of Dynein to β-catenin may also tether microtubules to AJs [30] . On the other hand, during apico-basal division in Drosophila , inscutable (insc) links the aPKC–Par complex and AJs to Dynein motors in order to recruit astral microtubules to the apical domain [31] . Therefore either because Gα–LGN–NuMA is mislocated, because microtubules are directly recruited by β-catenin or because aPKC ectopically recruits Insc, enlarged AJs could anchor astral microtubules anywhere within the apical domain, creating inadequate inward forces that provoke epithelial invagination. sβ-Catenin-expressing neuroblasts remain as progenitors but unexpectedly, they proliferate less. This reduced proliferation is caused by an extension of the M phase, which might be indicative of difficulties in chromosome pairing and/or segregation. Development of solid tumours depend on the accumulation of genetic mutations that prompt cells to over-proliferate and to invade neighbouring structures, thus their persistence as progenitors coupled with inaccurate chromosome pairing/segregation will increase the chances of sβ-catenin-expressing neuroblasts of subsequently acquiring mutations, and may represent an oncogenic threat for these cells. The loss of cell polarity has been associated with increased invasiveness and hence, malignancy, and recent studies have uncovered the importance of polarity regulators on tumour initiation [32] . However, we now propose that cytological abnormalities that would rather cause cell hyper-polarization, can also create growth aberrations with oncogenic potential. Medulloblastoma is a highly malignant primary brain tumour that originates in the posterior fossa. Up to four distinct molecular subgroups of medulloblastomas can be defined by their specific mRNA expression signatures: the WNT, SHH, Group 3 and Group 4 (ref. 33 ). However, WNT-type medulloblastoma is the least aggressive of the four molecular groups of medulloblastomas [33] . Indeed, even WNT-type medulloblastomas with a large-cell/anaplastic histology maintain the good prognosis of the WNT group [34] . Moreover, sβ-catenin expression significantly increases survival in a Shh-sub-type mouse model of medulloblastoma [35] . In addition, a WNT sub-type mouse model of medulloblastoma (expresses sβ-catenin in the hindbrain) develops aberrant cell collections in the dorsal brainstem during the foetal period that rarely progress to invasive tumours, unless other genes as Tp53 are also mutated [36] . Notably, the cell collections observed in this mouse model share similarities with the masses induced by sβ-catenin expression in the chicken embryos. Thus, although more studies would be required to demonstrate that the masses observed in the chicken embryos are really pre-neoplastic and whether they can actually generate a malignant tumour, we would like to speculate that the same cellular anomalies that maintain sβ-catenin-expressing cells as progenitors in this masses could be contributing to the distinctive low malignancy of this type of medulloblastoma by reducing its proliferation and migration. Antibodies and chemicals The source and working dilution for WB and IHC of the antibodies used in this work, is listed next. The mouse monoclonal antibodies used were raised against: proliferating cell nuclear antigen (Santa Cruz, SC-56 ) 1:500; HuC/D (Molecular Probes, A21271 ) 1:500; β-Tubulin III/Tuj1 (Covance, MMS435P ) 1:500; β-Actin (Sigma, AC15) 1:10,000; β-catenin (Sigma, C7207 ) WB 1:2,000 IHC 1:200; ZO-1 (Invitrogen, 1A12 ) WB 1:1,000 IHC 1:200; Pax6 (DSHB) 1:500; and glyceraldehyde 3-phosphate dehydrogenase (Enzo, 1D4) 1:1,000. The rat monoclonal antibodies were raised against: BrdU (AbD-Serotec, BU1/75 ) 1:500; and N-cadherin (Invitrogen, NCD-2 ) WB 1:2,000 IHC 1:200. The rabbit polyclonal antisera were raised against: GFP, RFP, FLAG and HA (produced in our laboratory) WB 1:3,000 IHC 1:1,000; Sox2 (Invitrogen, 48-1400 ) 1:100; Phospho S10 Histone3 (PH3, Millipore, 06-570 )1:1,000; aPKCζ/λ (Santa Cruz SC-17781 ) WB 1:10,000 IHC 1:500; and Phospho T410/403 aPKCζ/λ (Cell Signaling, 9378 ) 1:200. Alexa- (WB: 1:7,000, IHC 1:1,000) and peroxidase (1:10,000)-labelled secondary antibodies were obtained from Molecular Probes and Pierce, respectively; BrdU was purchased from Sigma and Rhodamine-Phalloidin (1:200) from Invitrogen. Analysing the number of divisions using Violet cell tracer We assessed the average number of divisions of neural progenitors in vivo using the Violet cell tracer (CellTrace Violet Cell Proliferation Kit, Invitrogen), a cytoplasmic retention dye that becomes diluted as cells divide. The Violet cell tracer was injected into the neural tube lumen at the time of electroporation. Embryos were then recovered at 48 h.p.e., the neural tube was carefully removed and the cells were dissociated following a 10–15-min digestion in Trypsin–EDTA (Sigma). The fluorescence intensity of the Violet tracer was measured in viable dissociated electroporated GFP + cells in the 405/450 nm excitation/emission range on a Gallios flow cytometer. The data are presented as the mean CellTrace violet intensity±s.d. that was obtained from six embryos per experimental condition. Chick embryo in ovo electroporation Eggs from White-Leghorn chickens were incubated at 38.5 °C in an atmosphere of 70% humidity. Embryos were staged according to Hamburger and Hamilton (HH) [37] . Chick embryos were electroporated with Clontech-purified plasmid DNA (1-2 μg ml −1 ) in H 2 O with Fast Green (50 ng ml −1 ). Briefly, plasmid DNA was injected into the lumen of HH stage 10–12 neural tubes, electrodes were placed at either sides of the neural tube and electroporation was carried out using an Intracel Dual Pulse (TSS10) electroporator delivering five 50 ms square pulses of 20 V for HH-10 and 25 V for HH-12. Transfected embryos were allowed to develop to the specific stages, then dissected, fixed and processed for IHC or in situ hybridization. For BrdU labelling, 5 μg μl −1 BrdU was injected into the neural tubes 1 or 4 h before fixation. This protocol has been approved by the ethical committee of CSIC (Ministerio de Economia y Competitividad, Spain). DNA constructs All the DNA constructs used, except the TopFlash and TopRed reporters, were cloned by PCR into either the PiggyBac or pCIG plasmids, two GFP-expressing bicistronic vectors. Modulators of Tcf-dependent transcription consisted of the Tcf3-HMG box alone (Tcf3-HMGB) or fused to either the VP16 activator (VP16-Tcf3) or to the Engrailed repressor (EnR-Tcf3). Fluorescence-associated cell sorting Embryos were electroporated with control (pCIG) or β-catenin S33Y vectors at the stages indicated, and 24 or 48 h.p.e., a single-cell suspension was obtained after a 10–15-min digestion with Trypsin–EDTA (Sigma). At least three independent experiments (six embryos in each experimental condition) were analysed by FACS. Hoechst and GFP/RFP were determined by flow cytometry using a MoFlo flow cytometer (DakoCytomation, Fort Collins, Colorado, USA) and the cellular DNA content was analysed (Ploidy analysis) in single-fluorescence histograms using Multicycle software (Phoenix Flow Systems, San Diego, CA, USA). IHC and BrdU incorporation Embryos were fixed for 4 h (up to HH-20) or overnight (bigger than HH-20) at 4 °C in 4% paraformaldehyde and immunostaining was performed on vibratome (40 μm) sections following the standard procedures. For BrdU detection, sections were incubated in 2 N HCl for 30 min and then rinsed with 0.1 M Na 2 B 4 O 7 (pH 8.5). After washing in phosphate-buffered saline-0.1% Triton, the sections were incubated with the appropriate primary antibodies and developed with Alexa- or Cyanine-conjugated secondary antibodies. After staining, the sections were mounted and examined on a Leica SP5 confocal microscope. Immunoblotting For immunoblotting experiments, both sides of the neural tube were electroporated sequentially. GFP+ areas of electroporated neural tubes were dissected under a fluorescence binocular microscope and after sonication, they were dissolved in 1 × SDS Laemmli sample buffer (five embryos per condition). The insoluble material was then removed by centrifugation and the samples were resolved by SDS–polyacrylamide gel electrophoresis (8% gels) and transferred to nitrocellulose membranes. The membranes were blocked with 8% non-fat dry milk in TTBS (150 mM NaCl, 0.05% Tween-20 and 20 mM Tris–HCl (pH 7.4)) and then incubated with the primary antibodies. The binding of the antibodies to the membranes was visualized with protein A/G-coupled peroxidase and using the ECL system, which was captured with the Versadoc Imaging System from Bio-Rad (N-cadherin) or Alexa-labelled secondary antibodies, which were detected with the Odyssey Infrared Imaging System from LI-COR (rest of the antibodies). The expression values were quantified with Quantity One software (Bio-Rad). Molecular weights were calculated using Bio-Rad Precision Molecular Weight Markers. Values were normalized with glyceraldehyde 3-phosphate dehydrogenase and the difference between control (pCIG) and β-catenin S33Y was calculated. The values shown represent the means±s.d. of three independent experiments. Full-gel scans are provided in Supplementary Fig. 10 . In vivo luciferase reporter assay Embryos were electroporated with the DNAs indicated together with a Sox2p luciferase reporter [14] , NeuroDp-Luciferase reporter [38] or with a 5 × Tcf-BS luciferase reporter construct containing synthetic Tcf-binding sites (TopFlash), as well as with a renilla construct (Promega) for normalization. GFP-positive neural tubes were dissected out at 48 h.p.e. and homogenized in passive lysis buffer. Firefly and renilla luciferase activity was measured by the Dual Luciferase Reporter Assay System (Promega), and the data are represented as the mean±s.d. from 12 embryos per experimental condition ( n >3). Quantitative fluorescence image analysis The relative amount of N-cadherin, ZO-1 and aPKC at the apical pole of β-catenin S33Y + cells was compared with the control-transfected neural tubes (pCIG). Confocal images were acquired using a laser-scanning confocal microscope (Sp5, Leica) and maximum projections of three consecutive confocal sections (2 μm total Z) were quantified with ImageJ software (National Institutes of Health). All images were converted into 32 bits, the background was subtracted and the original thresholds were set with the background as NaN (not a number). Finally, the mean grey value was quantified from an area containing the entire epithelial apical face. In total, 5–9 different images were used to calculate the mean value per embryo, and the bar graph represents the means±s.d. obtained from six different embryos per experimental condition. Cell sorting HH-12 chicken embryos were electroporated with sβ-catenin or control vector using PiggyBac system. Seven days post electroporation, the hindbrains were dissected (six per group), treated with trypsin–EDTA (Sigma-Aldrich) for 10–15 min to obtain a single-cell suspension and EGFP-positive cells separated with a cell sorter (FACS Aria III; BD). Reverse transcriptase real-time PCR Total RNA extracts were obtained following the TRIZOL protocol (Invitrogen) from sub-population of GFP+ cells (20,000 cells per pool). Reverse transcription and real-time PCR were performed according to the manufacturer’s instructions (Roche) using a lightcycler (LC 480; Roche). The sequence of the primers used for quantitative real-time –PCR amplification is indicated in Supplementary Table 1 . Oligonucleotides specific for chick glyceraldehyde 3-phosphate dehydrogenase were used for normalization. How to cite this article: Herrera, A. et al . Sustained Wnt/β-catenin signalling causes neuroepithelial aberrations through the accumulation of aPKC at the apical pole. Nat. Commun. 5:4168 doi: 10.1038/ncomms5168 (2014).